Alternative splicing modulates Kv channel clustering through a molecular ball and chain mechanism Ion channel clustering at the post-synaptic density serves a fundamental role in action potential generation and transmission. Here, we show that interaction between the Shaker Kv channel and the PSD-95 scaffold protein underlying channel clustering is modulated by the length of the intrinsically disordered C terminal channel tail. We further show that this tail functions as an entropic clock that times PSD-95 binding. We thus propose a ‘ball and chain’ mechanism to explain Kv channel binding to scaffold proteins, analogous to the mechanism describing channel fast inactivation. The physiological relevance of this mechanism is demonstrated in that alternative splicing of the Shaker channel gene to produce variants of distinct tail lengths resulted in differential channel cell surface expression levels and clustering metrics that correlate with differences in affinity of the variants for PSD-95. We suggest that modulating channel clustering by specific spatial-temporal spliced variant targeting serves a fundamental role in nervous system development and tuning. Voltage-activated potassium channels (Kv) are modular membrane proteins that play a fundamental role in action potential generation and transmission [1] . Although the shaping of action potentials relies on tight electro-mechanical coupling between the Kv channel membrane-spanning voltage sensor and ion conduction pore domains [2] , [3] , [4] , signal propagation along the axon and transmission across the synapse involves the cytoplasmic C-terminal tail [5] , [6] , [7] . The interaction of the tail segment of Kv channels with members of the synapse-associated protein family of scaffold proteins, such as the PSD-95 protein, underlies the precise localization, surface expression and clustering of many Kv channel molecules at the post-synaptic density (PSD) [7] , [8] , [9] . This interaction is responsible for prototypical Shaker Kv channel clustering at the fly neuromuscular junction and has been implicated in synaptic growth and plasticity [7] , [10] , [11] . Mechanistically, the interaction between the Kv channel tail and the PSD-95 scaffold protein underlying channel clustering is unique. It does not involve protein–protein interactions mediated by folded globular domains. Instead, as demonstrated for the prototypical Shaker B Kv channel variant, the interaction between the two proteins is mediated by a long and flexible intrinsically disordered segment of the channel tail carrying a short linear sequence motif at its tip able to bind the globular PDZ domains of PSD-95 (refs 12 , 13 ; see also refs 14 , 15 for reviews on intrinsically disordered proteins and their functions). Perturbations that change the intrinsically disordered nature of the Shaker B channel tail, in particular gross modifications that shorten the entire tail or affect its flexibility, or disruption of the canonical PDZ-binding motif were shown to affect scaffold protein binding [13] . Based on these observations, a fishing rod-like description of the interaction of the Kv channel and scaffold protein has been suggested, whereby disorder in the C-terminal tail of the channel would provide the orientational freedom needed for searching and finding the PSD-95 scaffold protein partner [13] . Given the stoichiometry of the interaction of the two proteins, dictated by the three consecutive PDZ interaction modules of PSD-95 and the four C-terminal tails of the oligomeric Kv channel, channel clustering results [16] . The fishing rod description of channel binding to scaffold protein suggests that C-terminal tail length modulates the Kv channel–PSD-95 interaction, in a manner reminiscent of the role of the N-terminal tail length on Kv channel fast inactivation, as described by the ‘ball and chain’ mechanism of Aldrich and co-workers [17] , [18] . Such an analogy is appealing, given that alternative RNA splicing of the Shaker Kv channel gene only occurs at those message segments that encode the N- and C-terminal tails, leading to the appearance of chains of different lengths [19] , [20] . One can thus ask whether alternative splicing at the C-terminal channel tail that yields the short and long Shaker A and B tail variants serves to modulate channel clustering, in particular in light of the fact that both tail variants carry exactly the same PDZ-binding motif at their end. The fact that spatial-temporal differences in the protein expression patterns of the two variants have been observed during development [21] , [22] , [23] points to the importance of C-terminal tail splicing in Kv channel physiology. To date, these spatial-temporal differences and their potential contribution to electrical signalling, in particular to synapse growth and plasticity, have been viewed through the lens of the observed differences in slow inactivation of the two versions of the Kv channel [21] , [22] . These differences, however, have been attributed to a single amino-acid difference within the sixth TM helix [24] , thus ignoring the potential role(s) of the different lengths of the A and B C-terminal tails in channel clustering. Does Kv channel clustering indeed occur according to a ‘ball and chain’ mechanism? As realized by Aldrich and co-workers in the 1990 (ref. 17 ) and later rephrased by Dunker and colleagues [14] , [15] using current terminology, two principal requirements must be met for such a binding mechanism to be valid. First, one must show that the underlying binding reaction is entropy controlled, as determined by chain length, and second, that chain length times protein complex formation. Thus, a ‘ball and chain’ sequence functions as an entropic clock [14] , [25] . Addressing these requirements in the context of the Kv channel–PSD-95 interaction requires thermodynamics, kinetics and energetic information, none of which is yet available. With the splicing-based channel clustering modulation hypothesis in mind, we examined how chain properties of natural or artificial short and long Kv channel tails affected k a , k d , K D , Δ S , Δ H and Δ G of the interaction of the channel with PSD-95 PDZ domains. Our results demonstrate that the Kv channel tail indeed functions as an entropic clock, thus encoding a C-terminal ‘ball and chain’ mechanism for Kv channel clustering. We show that the alternative splicing which leads to Shaker Kv channel C-terminal tail variability also gives rise to distinct channel affinities to PSD-95 and to distinct channel surface expression levels and cluster area size phenotypes. The implications of our results for electrical signalling, for PDZ-based protein–protein interactions and for the roles of intrinsically disordered proteins are discussed. The Kv channel tail is an entropic chain To address whether the Kv channel–PSD-95 interaction is entropy controlled, we took a reductionist approach and addressed how variations in channel tail length, either natural or artificial, affect the interaction with PSD-95 using surface plasmon resonance (SPR; Methods). 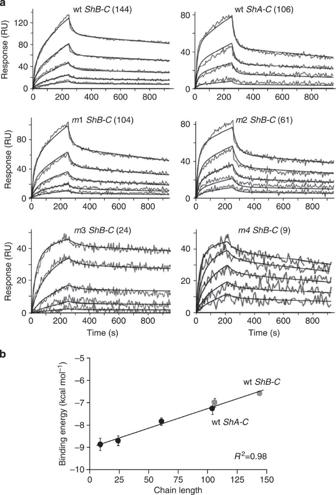Figure 1: TheShakerKv channel tail is an entropic chain that modulates PSD-95 binding. (a) SPR sensograms describing the association of PDZ2with wild-type and length-modifiedShB-Ctails (m1 to m4 deletion mutants) and with theShaker Anatural splice variant. Solid curves correspond to the thread lines obtained by global fitting of the data to a modified Langmuir isotherm describing protein–protein association kinetics (Methods). Values forkaandkdrate constants, respectively, determined from the association and dissociation phases, and for the corresponding equilibrium constant (KD), are reported inTable 1. (b) Plot of the association binding energy between natural and artificially shortenedShakertails indicated in A and PDZ2(−RTlnKA, seeTable 1) as a function of tail length. The solid curve corresponds to a linear regression with aR2correlation coefficient of 0.98. The wild-typeShA-CandShB-Ctails are indicated by grey symbols. All experiments were repeated three to five times and were performed at 25 °C. Figure 1a presents typical SPR sensograms describing the interaction of the second PDZ domain of PSD-95 (PDZ 2 ) with isolated natural Shaker A and B C-terminal tails (Δ ShA-C and ShB-C , respectively, comprising 106 and 144 residues) and with artificially shortened ShB-C chains 104, 61, 24 and 9 residues in length, all having the terminal PDZ-binding motif (Methods). As can be seen, for all interaction examined, clear time-dependent association and dissociation phases are apparent. Furthermore, and as expected, the association phase is found to be concentration dependent. Sensograms of each channel tail (at all concentrations tested) were globally fitted to a modified Langmuir isotherm describing a widely accepted protein–protein association model involving encounter complex formation followed by an induced fit rearrangement step [26] (Methods), and as previously demonstrated for interactions involving PSD-95 PDZ domains [27] . Estimates for the association and dissociation rate constants ( k a and k d ) of the interactions between PDZ 2 and the different tail variants, as well as the corresponding equilibrium constant ( K D ) are listed in Table 1 . Examining the steady-state properties of the Kv channel tail interaction with PDZ 2 revealed a linear correlation between the association binding energy of the two proteins and Kv channel chain length ( Fig. 1b ; R 2 =0.98), with a slope of 0.018 kcal mol −1 /residue. Thus, the shorter is the Kv channel chain, the higher is the affinity for PDZ. In particular, the short tail A splice variant exhibited higher affinity for PDZ 2 than did the long tail B variant. The short tail A splice variant further exhibited almost identical affinity for PDZ 2 as did the ShB-C chain variant artificially shortened to a similar size (106 and 104 amino acids, respectively). The length modulation of the tail–PDZ interaction was further shown using a pull-down experimental setup that mimics the native membrane context of the channel ( Supplementary Note 1 and Supplementary Fig. 1 ). Furthermore, the observation that the intrinsically disordered ShB-C chains, as well as the ShA-C chain, affect PSD-95 binding in a coherent manner suggests that the short tail A variant is also intrinsically disordered, as indeed verified using a variety of biophysical and spectroscopic approaches ( Supplementary Note 2 and Supplementary Fig. 2 ). Figure 1: The Shaker Kv channel tail is an entropic chain that modulates PSD-95 binding. ( a ) SPR sensograms describing the association of PDZ 2 with wild-type and length-modified ShB-C tails (m1 to m4 deletion mutants) and with the Shaker A natural splice variant. Solid curves correspond to the thread lines obtained by global fitting of the data to a modified Langmuir isotherm describing protein–protein association kinetics (Methods). Values for k a and k d rate constants, respectively, determined from the association and dissociation phases, and for the corresponding equilibrium constant ( K D ), are reported in Table 1 . ( b ) Plot of the association binding energy between natural and artificially shortened Shaker tails indicated in A and PDZ 2 (− RT ln K A , see Table 1 ) as a function of tail length. The solid curve corresponds to a linear regression with a R 2 correlation coefficient of 0.98. The wild-type ShA-C and ShB-C tails are indicated by grey symbols. All experiments were repeated three to five times and were performed at 25 °C. Full size image Table 1 Rate and equilibrium constants for the Shaker Kv channel tail–PSD-95 interaction*. Full size table Our results can be rationalized by considering the entropic contribution of the binding reaction; shorter chains lose less entropy upon binding than do longer chains as the configurational entropy of the latter is restricted to a greater extent upon binding [13] , [28] . Our findings thus argue that the A and B tail splice variants are pure entropic (random) chains, the lengths of which determine affinity for the scaffold protein partner. The Kv channel tail is an entropic clock To examine whether the channel tail functions as an entropic clock [14] , [25] able to time complex formation, we compared the kinetics of association and dissociation of the different channel tails to PDZ 2 ( Fig. 2 ). The normalized SPR response of all artificial and natural Shaker chains as a function of time at identical chain concentrations (2 μM) revealed that differences between the chains are seen only during association; only minor changes in the dissociation kinetics of the different tail–PDZ 2 complexes were observed over time ( Fig. 2a ). Furthermore, the shorter the chain, the faster were the association kinetics. In particular, the association kinetics of the A tail to PDZ 2 is faster than that of the B natural tail variant. The kinetics behaviour observed in Fig. 2a is, moreover, independent of chain concentration and is further reflected in the values of the k a and k d rate constants ( Table 1 ). As can be seen in the log k d versus log k a plot ( Fig. 2b ), no dependence between the two rate constants is seen. Whereas k a values for the longer and shorter channel chains vary by almost three orders of magnitude, protein dissociation once the complex has formed is independent of chain length, as revealed by the similar k d values obtained for all chains. This latter outcome is expected, considering that all shortened chains bear the same PDZ domain recognition motif. The chain length-dependent k a -only effects further imply that the Kv channel tail presents a native-like position in the transition state of Kv channel–PSD-95 association, as indeed verified using linear free energy relations adapted from physical organic chemistry ( Supplementary Note 3 and Supplementary Fig. 3 ). Taken together, our results argue that the Shaker Kv channel C-terminal tail is an entropic clock, the length of which times channel and scaffold protein complex formation. 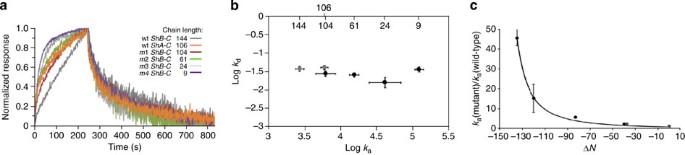Figure 2: TheShakerchannel tail is an entropic clock that times scaffold protein binding. (a) Comparison of the normalized association and dissociation kinetics of the natural and length-modified tail variants to and from PDZ2. For each trace, identical concentrations of PDZ2andShA/B-Ctails were used and the curve was normalized relative to the maximal response at the end of the association phase. (b) Association–dissociation rate constant correlation plot of theShA/B-C–PDZ2interaction. Values for the wild-type and mutant rate constants are indicated inTable 1. The wild-typeShA-CandShB-Ctails are indicated by grey symbols. Numbers on the upper horizontal axis indicate tail chain length. (c) Dependence of the scaledShA/B-C-PDZ2association rate constant (kamutant/kawild type ΔShB)) on chain length difference (ΔN). The solid line represents the best fit of the data to equation (1) (see text) describing a random flight ‘ball and chain’ mechanism for channel tail binding to PDZ2. The values for the wild-typeShA-CandShB-Ctails are indicated by grey symbols. Figure 2: The Shaker channel tail is an entropic clock that times scaffold protein binding. ( a ) Comparison of the normalized association and dissociation kinetics of the natural and length-modified tail variants to and from PDZ 2 . For each trace, identical concentrations of PDZ 2 and ShA/B-C tails were used and the curve was normalized relative to the maximal response at the end of the association phase. ( b ) Association–dissociation rate constant correlation plot of the ShA/B-C –PDZ 2 interaction. Values for the wild-type and mutant rate constants are indicated in Table 1 . The wild-type ShA-C and ShB-C tails are indicated by grey symbols. Numbers on the upper horizontal axis indicate tail chain length. ( c ) Dependence of the scaled ShA/B-C -PDZ 2 association rate constant ( k a mutant/ k a wild type Δ ShB )) on chain length difference (Δ N ). The solid line represents the best fit of the data to equation (1) (see text) describing a random flight ‘ball and chain’ mechanism for channel tail binding to PDZ 2 . The values for the wild-type ShA-C and ShB-C tails are indicated by grey symbols. Full size image To learn more on the mechanism underlying the regulation of the PSD-95–channel association by chain length, we plotted the ratio of association rate constants for mutant and wild-type channel tails (natural or artificial) as a function of chain length difference (Δ N ; Fig. 2c ), in a manner analogous to the approach used to study the relation between inactivation rate constants and chain lengths for the fast (N-type) inactivation of this channel [29] . As there, monotonic power law dependence for the association rate constant ratio on Δ N is observed. The data were fitted to the following theoretical ‘random walk’-based equation, derived assuming a pure ‘ball and chain’ mechanism: where k a (m) and k a (wt) correspond to the respective deletion mutant and wild-type (Δ ShB-C ) association rate constants and N to chain length. In deriving this equation, the chain is assumed to be devoid of any structure and to function as an entropic coil seeking the receptor site [29] . As can be seen in Fig. 2c , the data are adequately fitted to equation (1) ( R 2 =0.96), yielding estimates for the power law dependence ( n ) and for chain length ( N ) of 1.56 (±0.10) and 149 (±4), respectively. The estimated n value is almost identical to the 3/2 theoretical power law value expected for a pure ‘ball and chain’ mechanism. Furthermore, the chain length estimated here only slightly differs from the actual size of the 144 amino acid-long wild-type ShB-C reference chain. The Kv channel tail–PSD-95 interaction is entropy controlled The SPR results above suggest that the Kv channel tail–PSD-95 interaction is entropy controlled. This inference is, however, based on indirect measurements. Therefore, to directly address the role of entropy in modulating the Kv channel–PSD-95 interaction, we took advantage of our reductionist approach involving isolated soluble proteins and employed isothermal titration calorimetry (ITC) to evaluate the entropy (Δ S ), enthalpy (Δ H ) and Gibbs free-energy (Δ G ) changes that occur upon association of length-modified channel tails with PDZ 12 (corresponding to the first two PDZ domains of PSD-95). The ITC setup involves soluble proteins and as such is not best mimic of the native context of a membrane-bound channel. However, as will be delineated below, it enables obtaining valuable information that cannot otherwise be estimated. In the ITC experiments, the 104, 61, 24 and 9 residue-long ShB-C tails were studied since only they exhibit relatively high affinity for PDZ domains as required for reliable ITC measurements. All four ShB-C tails generated ITC titration curves reflecting the heat released at each injection as a function of the PDZ 12 /tail molar ratio, thus allowing for reliable thermodynamic parameter extraction ( Fig. 3a ). Fitting the titration binding curves to a simple Langmuir binding isotherm yielded reliable estimates of Δ H , T Δ S and Δ G of PDZ 12 -Kv channel tail association, as reported in Table 2 and further analysed in Fig. 3b–f . First, for all four chain-PDZ 12 pairs, Δ H of association was found to be almost identical and to contribute favourably to Δ G , as reflected by the negative sign of Δ H ( Fig. 3b and Table 2 ). Second, all four reactions exhibited unfavourable entropy changes upon association (indicated by the negative sign for T ΔS; Table 2 ), as expected for binding reactions involving entropic random chains. Moreover, the entropy changes seen upon ShB-C tail-PDZ 12 association linearly depend on chain length, with the shortest chain making a less unfavourable contribution to Δ G of association, as compared with longer chains ( Fig. 3c ). Third, Δ H shows no dependence on T Δ S , that is, no enthalpy-entropy compensation is observed for the tail-PDZ 12 association ( Fig. 3d ). Fourth, the free energy of tail–PDZ domain associations derived from the ITC measurements are linearly correlated with those estimated by SRP ( Fig. 3e ). As different PSD-95 PDZ fragments were used in each assay (PDZ 12 versus PDZ 2 ), this, together with the SPR data presented in Fig. 1b , demonstrates that tail length modulation of the Kv channel–PSD-95 interaction is insensitive to the PSD-95 PDZ fragment used. The different PDZ domain Kv channel partners may further rationalize differences in absolute affinity values seen in both analyses (compare Tables 1 and 2 ) [8] . Finally, the association rate constants and Δ S values obtained from both SPR and ITC measurements are as well linearly correlated ( Fig. 3f ). Taken together, the ITC results demonstrate in a direct manner that the Kv channel tail–PSD-95 interaction is entropy controlled. 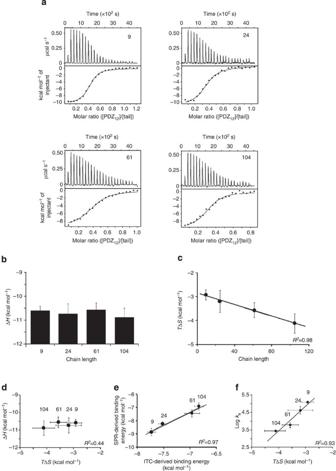Figure 3: The Kv channel tail–PSD-95 interaction is entropy controlled. (a) ITC titrations of Kv channel tail binding to PDZ12monitors changes in heat released as a function of analyte injection. PDZ12binding to fourShB-Ctail variants, 9, 24, 61 and 104 residues in length, was evaluated. The ITC-derived binding curves, describing the integrated heat released in each injection as a function of the molar ratio between the channel tail and the PDZ12protein, are shown below each panel. (b) The enthalpy change (ΔH) upon channel tail binding to PDZ12is constant and invariant of chain length. (c) The dependence of the entropy change (TΔS) upon tail-PDZ12association on chain length evaluated at 25 °C. (d) Enthalpy-entropy correlation plot of theShB-C–PDZ12interaction. (e) Correlation plot relating the Gibbs binding energy of the channel tails indicated in A to the PDZ domains of PSD-95 as estimated by SPR and ITC analyses. The solid curve corresponds to a linear regression with aR2correlation coefficient of 0.95. Note that different PSD-95 PDZ fragments were used in the SPR and ITC analyses (PDZ2and PDZ12, respectively). (f) Correlation plot relating the entropy change (TΔS) and association rate constant (ka) of tail binding to PDZ domains of PSD-95, as, respectively, estimated by SPR and ITC analysis. All experiments were repeated three times and were performed at 25 °C. Figure 3: The Kv channel tail–PSD-95 interaction is entropy controlled. ( a ) ITC titrations of Kv channel tail binding to PDZ 12 monitors changes in heat released as a function of analyte injection. PDZ 12 binding to four ShB-C tail variants, 9, 24, 61 and 104 residues in length, was evaluated. The ITC-derived binding curves, describing the integrated heat released in each injection as a function of the molar ratio between the channel tail and the PDZ 12 protein, are shown below each panel. ( b ) The enthalpy change (Δ H ) upon channel tail binding to PDZ 12 is constant and invariant of chain length. ( c ) The dependence of the entropy change ( T Δ S ) upon tail-PDZ 12 association on chain length evaluated at 25 °C. ( d ) Enthalpy-entropy correlation plot of the ShB-C –PDZ 12 interaction. ( e ) Correlation plot relating the Gibbs binding energy of the channel tails indicated in A to the PDZ domains of PSD-95 as estimated by SPR and ITC analyses. The solid curve corresponds to a linear regression with a R 2 correlation coefficient of 0.95. Note that different PSD-95 PDZ fragments were used in the SPR and ITC analyses (PDZ 2 and PDZ 12 , respectively). ( f ) Correlation plot relating the entropy change ( T Δ S ) and association rate constant ( k a ) of tail binding to PDZ domains of PSD-95, as, respectively, estimated by SPR and ITC analysis. All experiments were repeated three times and were performed at 25 °C. Full size image Table 2 Thermodynamic parameters of the K v channel tail PSD-95 interaction*. Full size table Distinct surface expression levels of the Kv channel variants We next examined whether the differences in the affinities of Kv channel natural variants to PSD-95, seen at the molecular level, are also reflected in the cellular context. Channel cell surface expression was first examined by transfecting embryonic Drosophila Schneider cells to express the isolated Shaker A or B tails fused to the CD8 membrane-targeting sequence, either alone or along with a PSD-95–GFP fusion protein, as described before [13] . Cell surface expression was assessed by confocal microscopy. Typical images for each case are presented in Fig. 4 . Control experiments showed that the PSD-95–GFP fusion protein is expressed throughout the cytoplasm ( Fig. 4a , left panel) and that cells expressing either the Shaker A or B tails alone showed homogeneous protein expression along the plasma membrane (PM), as revealed using anti-CD8 antibodies ( Fig. 4a , middle and right panels, respectively). Expression of PSD-95–GFP and of the either Shaker A or B channel tails ( Fig. 4b,c , respectively) resulted in changes in tail membrane surface expression and in PSD-95 membrane association, as respectively reflected in the red Shaker A or B tail-associated fluorescence pattern, reflecting the binding of antibodies to the CD8 tag (left columns) and the green PSD-95–GFP-based fluorescence pattern detected at the cell edge (middle columns). The yellow colouring of the merged images (right columns) shows overlap of PSD-95 and the A and B channel tails, reflecting protein co-localization. Thus, the interaction between the two proteins can be detected in vivo . Clear differences in cell surface expression pattern are, however, observed in each case. The long tail, lower affinity B channel variant is less well expressed in the cell membrane than is the shorter high-affinity A variant (compare panels 4b and c). This is due, in part, to PSD-95-mediated redistribution of the tail to endosome-like structures that preferentially hamper membrane cell surface expression of the B variant. Less of the A tail is redistributed to such structures, with the majority reaching the cell surface. The effects were quantified by evaluating the average fractional co-localization of PSD-95 with either the A and B tails at the membrane surface and in internal membrane compartments ( n =12–13 cells; Methods). Although, in the case of the A short tail variant the fractional PSD-95-mediated PM expression was around 90%, only 60% of the long-tail B variant co-localized to the PM ( P -value <0.01; Fig. 4d ). The results are thus coherent with the reported role of PSD-95 in stabilizing the Kv channel at the membrane surface as achieved by chaperoning more copies of the channel to the cell PM [7] , [8] and upon suppressing endocytosis-mediated channel internalization [30] . 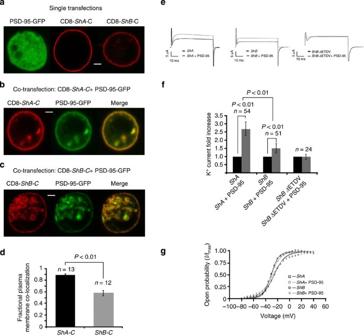Figure 4: TheShaker AandBspliced variants exhibit distinct cell surface expression levels. (a) Confocal microscopy analysis of DrosophilaS2 Schneider cells expressing PSD-95–GFP or either of theShaker AandBtails fused to the CD8 membrane-targeting sequence. (b,c) Confocal microscopy analysis ofDrosophilaS2 Schneider cells co-expressing PSD-95–GFP and either the CD8-ShA-C(b) or CD8-ShB-Cvariant (c). For each cell, three images are shown, with the red channel-associated and green PSD-95-associated fluorescence signals presented in the left and middle columns, respectively. The merged image of each cell is given in the right-most column. Scale bars in panelsa–ccorrespond to 2 μm. (d) Differences in PSD-95-mediated membrane surface expression of theAandBchannel tails (Methods) are statistically significant based on a Student’st-test (n=12–13;P<0.01). (e) K+current expression levels of the full-lengthShaker AandBchannel variants and of theBchannel variant lacking the terminal PDZ-binding motif (ΔShB-C-ΔETDV) recorded from oocytes injected with mRNA encoding either variant with or without PSD-95 mRNA. K+currents were elicited by applying a +40 mV depolarizing pulse from a holding potential of −85 mV (Methods). (f) Statistical analysis of PSD-95-mediated fold increase in potassium current level expression of theShaker AandBvariants (n=~50). Differences in current expression were found to be statistically significant based on a Student’st-test and considering Bonferroni’s correction for multiple comparisons (based on aP-value lower than 1%). (g) Open probability (I/Imax) curves of theShaker AandBchannel variants in the presence or absence of PSD-95. Smooth curves correspond to a two-state Boltzmann gating isotherm. The values for the half activation voltage (V1/2) and activation slope (Z) gating parameters of theShaker AorBvariants, in the presence or absence of PSD-95, are listed inSupplementary Table 1. Error bars in the appropriate figure panels represent s.e.m. values. Figure 4: The Shaker A and B spliced variants exhibit distinct cell surface expression levels. ( a ) Confocal microscopy analysis of D rosophila S2 Schneider cells expressing PSD-95–GFP or either of the Shaker A and B tails fused to the CD8 membrane-targeting sequence. ( b , c ) Confocal microscopy analysis of Drosophila S2 Schneider cells co-expressing PSD-95–GFP and either the CD8- ShA-C ( b ) or CD8- ShB-C variant ( c ). For each cell, three images are shown, with the red channel-associated and green PSD-95-associated fluorescence signals presented in the left and middle columns, respectively. The merged image of each cell is given in the right-most column. Scale bars in panels a – c correspond to 2 μm. ( d ) Differences in PSD-95-mediated membrane surface expression of the A and B channel tails (Methods) are statistically significant based on a Student’s t -test ( n =12–13; P <0.01). ( e ) K + current expression levels of the full-length Shaker A and B channel variants and of the B channel variant lacking the terminal PDZ-binding motif (Δ ShB-C -ΔETDV) recorded from oocytes injected with mRNA encoding either variant with or without PSD-95 mRNA. K + currents were elicited by applying a +40 mV depolarizing pulse from a holding potential of −85 mV (Methods). ( f ) Statistical analysis of PSD-95-mediated fold increase in potassium current level expression of the Shaker A and B variants ( n =~50). Differences in current expression were found to be statistically significant based on a Student’s t -test and considering Bonferroni’s correction for multiple comparisons (based on a P -value lower than 1%). ( g ) Open probability ( I/I max ) curves of the Shaker A and B channel variants in the presence or absence of PSD-95. Smooth curves correspond to a two-state Boltzmann gating isotherm. The values for the half activation voltage ( V 1/2 ) and activation slope ( Z ) gating parameters of the Shaker A or B variants, in the presence or absence of PSD-95, are listed in Supplementary Table 1 . Error bars in the appropriate figure panels represent s.e.m. values. Full size image The results above demonstrate a correlation between the in vitro and in vivo binding studies, both performed using a reductionist approach involving only the isolated channel tails. To address the effect of PSD-95 in mediating the membrane expression of the A and B tails at the whole channel level, electrophysiology recordings were collected (Methods), as previously described for the NMDA receptor protein [31] . In such measurements, the potassium current level of Kv channel-expressing Xenopus laevis oocytes directly reflects the membrane surface expression of properly assembled functional channels. Figure 4e presents the voltage-induced changes in K + current level seen upon co-expressing either of the A and B Shaker variants with PSD-95. As can be seen, oocytes co-injected to express either of the Shaker A and B channels along with PSD-95 revealed higher K + current levels, as compared with the case where only channel cRNA was injected. In each case, the observed fold increase in current density is statistically significant, as evaluated from a Student’s t -test ( n =~50; P -value <0.01). No difference was observed for oocytes expressing the PSD-95 protein along with a B channel variant lacking the last four terminal PDZ-binding motif residues (Δ ShB-C -ΔETDV). Moreover, the fold increase in current density recorded for the Shaker A channel was close to twofold higher than that of the B channel ( P -value <0.01; Fig. 4f ), in agreement with the results reported above ( Fig. 4d ). The observed differences in cell surface expression level of the two channel variants are not the result of changes in channel open probability as the activation curves of both the A and B channel variants in the presence or absence of PSD-95 are similar ( Fig. 4g ). This is further revealed upon assessment of the Z and V 1/2 characteristic gating parameters of the four curves using a Boltzmann gating isotherm, all found to be similar ( Supplementary Table 1 ). Taken together, our results obtained using both reductionist and whole channel setups are coherent and suggest that PSD-95 is able to chaperone more copies of the short-tail high-affinity A channel variant to the cell membrane, as compared with the long-tail low-affinity B variant. Distinct clustering phenotypes of the Kv channel variants Next, we addressed whether the A and B natural channel variants also exhibit differences in PSD-95-mediated Kv channel clustering. This question is best answered using analysis at the whole channel level so as to ensure that the proper stoichiometry needed to attain channel clusters [16] . We thus transfected Drosophila Schneider cells to express the full-length Shaker A or B channels fused to a cherry fluorescence marker, either alone or along with a PSD-95–GFP fusion protein. Typical confocal microscopy images for each case are presented in Fig. 5 . Control experiments involving cells transfected to express either of the full-length Shaker A or B channels alone showed no localization of either at the PM ( Fig. 5a ). Instead, the two channel variants were detected throughout the cytoplasm, with a slightly denser distribution seen in the nuclear membrane. No difference was observed in the expression patterns of the two channel variants when introduced alone. However, co-expression of PSD-95–GFP and either of the Shaker A or B channel variants ( Fig. 5b,c , respectively) resulted in channel membrane surface expression and clustering and in PSD-95-membrane association, as, respectively, reflected in the red Shaker A or B channel-associated fluorescence (left columns) and the green PSD-95–GFP-based fluorescence pattern (middle columns). The membrane-associated yellow colouring of the merged images (right columns) shows overlap of PSD-95 and the A and B channel tails, reflecting the protein co-localization underlying channel surface expression and clustering. Prominent differences were observed in each case. Whereas the B channel clustering presented a speckled pattern of small-sized clusters, more extensive clustering was observed with the A variant, with the clusters being of much bigger size (the A and B variants co-localization images are of similar scale). The effects were quantified by examining the metrics of PSD-95-mediated A or B channel cluster formation using ~12–16 different cells for each variant (Methods). Overall, ~270 and 160 clusters were analysed for the A and B channel variants, respectively. The results, comparing the average number of clusters per cell, average cluster area size and distribution of cluster area sizes of the two variants are presented in Fig. 5d–f , respectively. The analysis revealed that no significant difference was observed in the averaged number of clusters per cell between the A and B variants, found to be 16.3 (±1.1) and 14.0 (±1.4), respectively ( Fig. 5d ). Second, the average cluster area size of the A channel variant was greater by ~40% than that of the B channel variant ( Fig. 5e ; P <0.01 by a Wald χ 2 test (Methods)). Moreover, as can be seen in Fig. 5f , the distributions of cluster area sizes of the two variants had different shapes and ranges, with that of the A variant being skewed towards larger cluster area sizes. Statistical validation of these differences were performed by Kolmogorov–Smirnov and Moses extreme reaction tests, respectively (Methods), with P <0.01 for both tests. Taken together, these results reveal that, whereas no differences were observed in the average number of variant clusters per cell, the short-tail high-affinity A channel variant supports clusters of larger area than does the long-tail low-affinity B channel variant, thus rationalizing the observed differences in cell surface expression between the two ( Fig. 4 ). 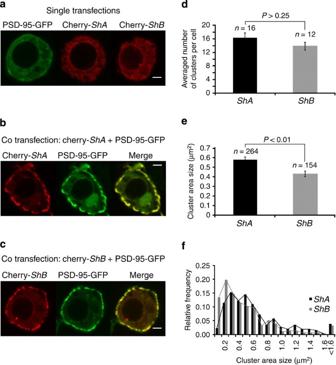Figure 5: TheShaker AandBvariants exhibit differences in cluster area size. (a) Confocal microscopy analysis ofDrosophilaS2 Schneider cells expressing PSD-95–GFP or either of the full-lengthShaker AandBchannels fused to the mCherry fluorescent marker (Methods). (b,c) Confocal microscopy analysis ofDrosophilaS2 Schneider cells co-expressing PSD-95–GFP and either the mCherry-ShAvariant (b) or mCherry-ShBvariant (c). For each cell, three images are shown, with the red channel-associated and green PSD-95-associated fluorescence signals presented in the left and middle columns, respectively. The merged image of each cell is shown in the right column. Scale bars ina–ccorrespond to 2 μm. (d) Comparison of the average number of plasma membrane-associatedAandBchannel clusters per cell (n=~12–16;P>0.25 in Student’st-test). (e) Comparison of averaged area size ofAandBchannel clusters (n=150–260;P<0.01 in Waldχ2test (see Methods)). (f) Cluster area size distribution of theAandBchannel variants, as supported by PSD-95. Distributions in steps of 0.1 μm2are presented. For clarity, the peaks of each bar are linked. Error bars in the appropriate figure panels represent s.e.m. values. Figure 5: The Shaker A and B variants exhibit differences in cluster area size. ( a ) Confocal microscopy analysis of Drosophila S2 Schneider cells expressing PSD-95–GFP or either of the full-length Shaker A and B channels fused to the mCherry fluorescent marker (Methods). ( b , c ) Confocal microscopy analysis of Drosophila S2 Schneider cells co-expressing PSD-95–GFP and either the mCherry- ShA variant ( b ) or mCherry- ShB variant ( c ). For each cell, three images are shown, with the red channel-associated and green PSD-95-associated fluorescence signals presented in the left and middle columns, respectively. The merged image of each cell is shown in the right column. Scale bars in a – c correspond to 2 μm. ( d ) Comparison of the average number of plasma membrane-associated A and B channel clusters per cell ( n =~12–16; P >0.25 in Student’s t -test). ( e ) Comparison of averaged area size of A and B channel clusters ( n =150–260; P <0.01 in Wald χ 2 test (see Methods)). ( f ) Cluster area size distribution of the A and B channel variants, as supported by PSD-95. Distributions in steps of 0.1 μm 2 are presented. For clarity, the peaks of each bar are linked. Error bars in the appropriate figure panels represent s.e.m. values. Full size image Our results argue that the Kv channel-scaffold protein interaction is entropy controlled and further demonstrate that the length of the Kv channel tail times complex formation with the PSD-95 partner. The Kv channel tail thus functions as an entropic clock and encodes a C-terminal ‘ball and chain’ mechanism for Kv channel binding to scaffold proteins that is analogous to the N-terminal ‘ball and chain’ mechanism describing channel fast inactivation ( Fig. 6 ) [17] , [18] . Several lines of evidence support the analogy between the two N- and C-terminal ‘ball and chain’ mechanisms. First, the seminal studies of Hoshi et al . [17] on fast channel inactivation clearly showed dependence of the inactivation process on chain length, arguing that this reaction is entropy controlled. This has been demonstrated for the Kv C-terminal channel segment as we have shown length-based modulation of Kv tail-PSD-95 affinity ( Figs 1b and 2c ) and further showed, in a direct manner, that length-dependent changes in the free energy of Kv channel tail–PDZ association are brought about by changes in entropy alone (Fig. 3c). Second, the earlier studies showed that the N-terminal channel tail acts as a molecular clock that times channel fast inactivation [14] , [17] , with the length of the segment determining the kinetics of entry to inactivation [29] . Our findings that Kv channel tail length only affects the kinetics of PDZ association ( k a ) but not dissociation ( k d ; Fig. 2a,b ) agree with findings of the Aldrich group and suggests a similar timing function for the C-terminal channel tail. Third, and along the same line, Jemth et al . presented complementary data showing that mutations in a PDZ-binding motif peptide, all producing variants of identical length, only affected the dissociation rate constant of the peptide from the PSD-95 PDZ domain ( k d ) without changing the association rate constant ( k a ) [32] . This result is in perfect agreement with a ‘ball and chain’ mechanism. Fourth, the power law dependence of the normalized association rate constant on tail length ( Fig. 2c ) is adequately explained by a random walk ‘ball and chain’ theory (based on Flory’s seminal formulation [33] ), as also found for the dependence of the entry to inactivation rate constant in chain length [29] . Finally, the finding that alternative splicing in Shaker Kv channel mRNA only affects the N- and C-terminal tails to produce chains of different length [19] , [20] further strengthens the analogy between the ‘ball and chain’ mechanisms. 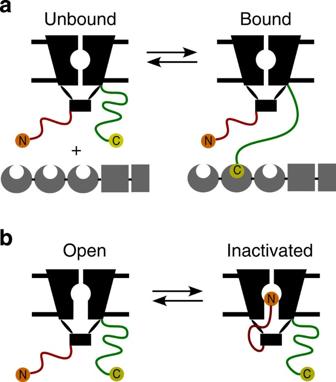Figure 6: A C-terminal ‘ball and chain’ mechanism for Kv channel binding to PSD-95. Schematic representation of the ‘ball and chain’ mechanisms for channel clustering (a) and fast inactivation (b). In the clustering intermolecular ‘ball and chain’ mechanism, K+channel recruitment of the PSD-95 scaffold protein is achieved upon binding of the chain-tethered C-terminal peptide ‘ball’ to PDZ domain(s) of PSD-95 in a precisely timed manner, based on the length of the Kv channel C terminal chain. In the intramolecular fast inactivation mechanism, the open channel pore (O) inactivates (I) in a precisely timed manner upon binding of the chain-tethered N-terminal peptide ‘ball’ to a receptor site within the inner cavity of the pore. The membrane-embedded portion corresponds to the channel voltage-sensor and pore domains, whereas the rectangular shape corresponds to the T1 domain. The crescent, box and rectangular shapes represent the PDZ, SH3 and guanylate kinase-like domains of the PSD-95 protein, respectively. Figure 6: A C-terminal ‘ball and chain’ mechanism for Kv channel binding to PSD-95. Schematic representation of the ‘ball and chain’ mechanisms for channel clustering ( a ) and fast inactivation ( b ). In the clustering intermolecular ‘ball and chain’ mechanism, K + channel recruitment of the PSD-95 scaffold protein is achieved upon binding of the chain-tethered C-terminal peptide ‘ball’ to PDZ domain(s) of PSD-95 in a precisely timed manner, based on the length of the Kv channel C terminal chain. In the intramolecular fast inactivation mechanism, the open channel pore (O) inactivates (I) in a precisely timed manner upon binding of the chain-tethered N-terminal peptide ‘ball’ to a receptor site within the inner cavity of the pore. The membrane-embedded portion corresponds to the channel voltage-sensor and pore domains, whereas the rectangular shape corresponds to the T1 domain. The crescent, box and rectangular shapes represent the PDZ, SH3 and guanylate kinase-like domains of the PSD-95 protein, respectively. Full size image One noteworthy difference exists, however, between the two mechanisms. Although the ball-receptor inactivation binding reaction is an intra-molecular process, the binding of the channel to PSD-95 is intermolecular and diffusion limited ( Fig. 6 ). This difference will affect the effective local concentration of the ‘ball’ near its receptor site and will be reflected in the magnitude and type of the forward binding rate constants, being first order for entry to inactivation and second order for tail–PDZ complex formation. However, considering that in the native context PSD-95 is a priori membrane-associated (because of its interactions with other membrane protein partners and its own plamitoylation [34] ) and the natural variation in Kv channel fast inactivation where the ‘ball and chain’ sequence is not carried on the channel itself but rather on the auxiliary β subunit with which it interacts [35] , the resemblance between the two inactivation and clustering ‘ball and chain’ mechanisms becomes even clearer. The analogy between the two ‘ball and chain’ mechanisms describing Kv channel activity is also noteworthy when considering the role(s) of intrinsically disordered protein segments, in general [15] , [25] . For both fast channel inactivation and channel binding to scaffold protein reactions, enthalpic and entropic contributions can be attributed to distinct sequence modules within the N- or C-terminal tails. Whereas the tail chain primarily controls the entropy of the binding reaction, as manifested by the dependence of k a and Δ S on chain length, the chain-tethered ‘ball’ (that is, the inactivation or PDZ-binding recognition motifs) primarily determines the enthalpy of the binding reaction, as manifested by the invariance of k d and Δ H as a function of chain length. We thus propose that the log k d –log k a and Δ H –Δ S profiles, in which the measured parameters show no dependence on each other upon changes in chain length ( Figs 2b and 3d , respectively), correspond to a thermodynamic signature of entropy controlled ‘ball and chain’ binding mechanisms involving entropic clocks. The nature of this signature is in contrast to the linear correlation between Δ H and Δ S often observed in structure-function studies of protein–protein interaction systems involving two globular proteins, a phenomenon referred to as enthalpy-entropy compensation [36] . The results presented here reporting protein tail length modulation of PDZ binding carry implications for PDZ-based protein–protein interactions, in general. Such interactions are of primary importance in protein interaction networks underlying a variety of cellular signalling processes [37] . It is generally assumed that the affinity of PDZ domains to their cognate proteins is solely determined by a short sequence motif composed of three to eight residues [37] , [38] . The observed affinities are typically within the sub-μM range [38] , affinities much higher than those measured here (μM range and higher ( Table 1 )). Such assertions were based on structural and functional studies involving isolated PDZ domains and model terminal PDZ-binding peptides and were aimed at deriving estimates for the affinity of the interaction and to reveal the minimal recognition motif important for binding [37] , [38] . However, long protein tails, often presenting an intrinsically disordered nature, usually flank terminal PDZ-binding motifs of membrane [12] and other proteins. To date, no rigorous assessment of protein tail length on interaction affinity has been reported. Our paper thus emphasizes that under certain circumstances, chain length plays an important role in mediating PDZ-based protein–protein interaction. In the case of the Kv channel, such tail length modulation considers the entropy contribution of random chains to PDZ domain binding, as predicted from polymer chain chemistry. Indeed, our longest Kv tail truncation, producing a nine amino-acid-long tail, reveals affinity in the sub-μM range ( Table 1 ), comparable to those values reported using model peptides [38] . We noted, however, that our reported association and dissociation rate constants for this tail are lower than those typically characterizing PDZ–peptide interactions [38] , a fact that may be related to the particular PDZ-Kv channel peptide interaction studied here. Although we cannot further explain this, the important point is that we focus here on relative chain length differences ( Fig. 2c ) [29] and thus, the observed length-dependent trends of the association rate and equilibrium constants are valid. We, therefore, propose that protein tail length may represent another dimension for controlling PDZ-based protein–protein interactions. Such modulation requires the tail to be a random chain, that is, a pure entropic chain. It is thus not surprising that the recently measured affinity of PDZ 2 for the 169 amino-acid-long intrinsically disordered tail of the NMDA receptor (NR2B) [39] , shown to be a non-random chain protein that undergo stochastic switching between distinct conformational states [40] , falls off the binding energy-length correlation presented in Fig. 1b ((x,y) NR2B-C =(169-7.8)). The conformity of the natural A and B tail variants with the entropic chain characteristics of the Kv–PSD-95 interaction, as manifested in the binding energy and association kinetics length profiles ( Figs 1b and 2c ), points to the physiological relevance of the C-terminal ‘ball and chain’ mechanism characterizing the Kv channel–PSD-95 interaction. Indeed, when assessed at both the tail alone and whole channel levels, the two variants exhibited distinct cell surface expression and clustering patterns that are coherent with the difference in affinity of the two variants, as rationalized by the ‘ball and chain’ mechanism. The high-affinity short-tail A variant presents higher cell surface expression level ( Fig. 4 ) and supports larger channel clusters in Schneider cell membranes than does the low-affinity long-tail B variant ( Fig. 5 ). Thus, molecular distinctions reflected in the differential interactions of the tail variants with PSD-95 translate into functional differences in the context of cellular channel clustering. The proposed ‘ball and chain’ mechanism for channel clustering sheds new light on the roles of the short A and long B tail variants in electrical signalling. We suggest that spatial and temporal differences in Shaker A and B expression during development [23] and/or channel variability resulting from hetero-oligomeric A and B subunit assembly [41] would give rise to distinct patterns of PSD-95-mediated A and B channel cell surface expression and clustering, in turn resulting in changes in channel current density at the post-synaptic site of homo- or hethero-oligomeric channel localization. This, subsequently, could lead to changes in action potential propagation and transmission, synaptic growth and plasticity. As such, it is tempting to speculate that a splicing-based developmental switch for the Shaker channel [23] is responsible for modulating channel clustering that may underlie changes in nervous system function and tuning during development. Although this appealing hypothesis requires further investigation, it is evident that the Shaker Kv channel protein system exemplifies how linkage between alternative splicing and intrinsic disorder enables functional diversity [42] . Molecular biology and protein expression and purification The PSD-95 protein used in the current study is the Drosophila S97 variant. Cloning of the C-terminal segment of the Shaker A channel variant (Δ ShA-C) into the His-tag-encoding pHis parallel vector was performed as described previously [13] , as was cloning of the second PSD-95 PDZ domain (PDZ 2 ) into the pET28a plasmid. The 144 amino-acid-long wild-type ShB-C tail was shortened to lengths of 104 (513–553) and 61 (Δ513–596) residues using looping out a Quick change mutagenesis kit (Stratagene). Deletion mutants of 24 (Δ513–633) and 9 (Δ513–648) residues were obtained using commercial peptide synthesis services. Peptides were purified to a degree greater than 98% and their concentrations were determined using standard analytical methods. A ShB-C tail 198 residue-long was achieved by triplicating a 27-amino-acid tail segment (580 to 607), predicted to be intrinsically disordered ( Supplementary Note 1 ). All constructs were verified by direct sequencing. For protein cell surface expression analysis, DNA coding for the tail of the Shaker A Kv channel spliced variant fused to the CD8 membrane-targeting sequence ( CD8-ShA-C ) was cloned into the Drosophila pUAST vector as previously described for the CD8-ShB-C variant [13] . For protein clustering analysis, DNA coding for the full-length Shaker A or B Kv channel variants was cloned into the Drosophila pUAST vector carrying the reading frame of the mCherry fluorescent protein marker. In both hybrid channel constructs, the mCherry marker was fused to the N terminal of the channel protein. All constructs were verified by sequencing of the entire gene. Expression and purification of ShB-C (or its tail deletions), ShA-C , PDZ 12 and PDZ 2 were performed as previously described [13] with the 6Hist tag removed as required for each pull down, ITS or SPR binding analyses. SPR analysis SPR was performed using a ProteOn XPR36 instrument (Bio-Rad). The PDZ 2 protein was bound to the mass-sensitive GLC chip by passing a solution of 50 μM PDZ 2 protein (total of 5 μg) in PBST buffer (pH 7.4) over the chip at a flow rate of 100 μl min −1 . Following binding and washing, different concentrations (0–50 μM) of the tail proteins in the same buffer were allowed to flow over the chip. Control experiments using BSA- or IgG-attached chips were performed and the resulting data were subtracted from the measured data. The PDZ 2 -tail binding experiments were repeated three to five times at 25 °C. Attaching the N-terminal end of the tail to a His tag chip was unsuccessful owing to nonspecific binding of the PDZ 2 protein to the chip and tail drifts during the experiment. Size exclusion chromatography For stokes radius determination, gel filtration of ShA-C and standard molecular weight marker proteins was performed on an analytic size exclusion column (Superdex 10/300), pre-equilibrated in buffer A (20 mM imidazole, 0.3 M NaCl, 50 mM Tris-HCl, pH 8) and run at a flow rate of 0.5 ml min −1 at room temperature on an AKTA FPLC system (Amersham-Pharmacia) [13] . The elution volumes of the standard and ShA-C proteins ( V e ) were converted into mobility factor parameters, K av, using the following equation: K av=( V e − V o )/( V t − V o ), where V o is the column exclusion volume (5.3 ml) and V t is the total column bed volume. The Stokes radius ( R ST ) of ShA-C was estimated using a linear calibration plot of R ST versus (−log K av) 1/2 , obtained with globular bovine proteins pancreatic ribonuclease A, chymotrypsinogen A, ovalbumin and serum albumin as standards. The theoretical Stokes radii of native ( R N ST ) or fully unfolded ( R RC ST ) proteins were determined as described by Uversky et al . [43] Analytical ultracentrifugation Equilibrium ultracentrifugation experiments were performed using a Beckman XL-A ultracentrifuge with an An60 Ti rotor at 20 °C, as previously described [13] . A concentrated sample of ShA-C was dialysed overnight against buffer A (20 mM imidazole, 0.3 M NaCl, 50 mM Tris-HCl, pH 8). Fractions of the sample were then diluted 1:2 and 1:3 with dialysate to generate final protein solutions of approximately 15, 31 and 63 μM, which were loaded into a six-sector cell and spun at rotor speeds of 19,000 and 21,000 r.p.m. Data were collected at each speed for each protein concentration at 230, 260, 280 and 320 nm and analysed using the following equation: M =[2 RT /(1−) ρω 2 ][(dln( c ))/d r 2 ], with set at 0.73 cm 3 g −1 and ρ at 1.012 g cm −1 , as calculated using Ultrascan software ( http://www.ultrascan.uthscsa.edu ) [13] . Circular dichroism (CD) spectroscopy CD wavelength scan measurements were recorded on a Jasco J-815 model CD spectrometer. All CD spectra were recorded in 10 mM NaCl, 5 mM Tris-HCl, pH 8, with a bandwidth of 2 nm and an averaging time of 1 s. Far-ultraviolet spectra were recorded at room temperature using a 1-mm cuvette and a ShA-C protein concentration of 0.25 mg ml −1 . Each spectrum presented is derived from ten independent spectra, averaged and baseline-corrected for the contribution of the sample buffer. 1 H-NMR spectroscopy NMR spectra were recorded in a 95% H 2 O/5% D 2 O solvent mixture. Data were acquired on a Bruker 500 MHz spectrometer and analysed with Bruker XWINNMR software. 1D- 1 H-NMR spectra were collected at room temperature, and water suppression was achieved using the WATERGATE sequence. Resolution enhancement was achieved by application of a sine-square window function to the free induction decay. Disorder prediction The intrinsic disorder tendency of ShA-C was calculated using the Foldindex disorder predictor ( http://bip.weizmann.ac.il/fldbin/findex ), based on the mean net charge and mean hydrophobicity properties of the sequence [43] , [44] . Predictions were further verified using the IUPred server ( http://iupred.enzim.hu/ ) [45] . Isothermal calorimetery ITC measurements were performed on a Nano-ITC instrument (TA Instruments, Microcalorimeter). The 9, 24, 61 and 104 amino-acid-long ShB-C tails at concentrations of 165, 200, 200 and 240 μM, respectively (in buffer containing 150 mM NaCl, 50 mM Tris-HCl, pH 8), were titrated by 23 injections of 2 μl buffer solution containing 650 μM of the PDZ 12 partner protein. Reference titrations were obtained by injecting PDZ 12 into cells containing buffer alone, with the heat of dilution being subtracted from the protein–protein titration data. The binding isotherms were best fitted to a simple independent model to yield the enthalpy change upon association and the association constant ( K A ) using NanoAnalyze Software (v2.4.1). Experimental errors in estimated parameters were derived using the software bootstrapping procedure for 1,000 trials and based on 95% confidence intervals. All experiments were carried out at 25 °C. Estimates of entropy changes upon tail–PDZ association were derived using the measured Δ H and Δ G values according to Δ G= Δ H−T Δ S. Confocal microscopy surface expression and clustering analyses Assessment of the membrane surface expression levels of the ShA-C and ShB-C Kv channel variants was performed essentially as previously described [13] . Briefly, Drosophila SR+ Schneider cells were transfected with the pUAST-CD8 -ShA-C or pUAST-CD8 -ShB-C plasmids either alone or with the pUAST-GFP-PSD-95 fusion plasmid, using the Escort IV system (Sigma). For immunostaining, ShA-C - or ShB-C -expressing cells were fixed and tail protein detection was performed using mouse anti-CD8 primary antibodies (BioLegend) followed by CY3-conjugated anti-mouse secondary (monoclonal) antibodies. PSD-95 detection was performed using the associated green GFP fluorescence signal. Cell images were taken using a LSM510 Zeiss confocal microscope. Assessment of channel clustering of the full-length A and B channel variants was performed by transfecting Schneider cells with pUAST-mCherry- ShA or pUAST-mCherry- ShB fusion plasmids either alone or with the pUAST-GFP-PSD-95 fusion plasmid. For examining channel clustering, cells were fixed and detection of fusion channel and PSD-95 proteins was performed using the respective associated red and green fluorescence signals. Cell images were taken at the equatorial focus plane, such that the nucleus exhibited its longest dimension. Electrophysiology K + currents were recorded from the Shaker A or B channels under conditions of two-electrode voltage clamp (OC725B, Warner Instruments) 1–3 days after injecting equal amounts of either Shaker A and B mRNA (50 ng) with or without PSD-95 mRNA [46] . Oocytes were held at a resting membrane voltage of (85 mV and K + currents were elicited upon a depolarizing step to +40 mV. Voltage-activation curves were obtained using a standard tail current protocol and represent the average of recordings from more than ten different oocytes. Care was taken to measure oocytes expressing K + tail currents in a narrow range of 2–5 μA. Data analysis SPR sensograms were globally fitted to the widely accepted two-step protein–protein association model involving an encounter complex formation followed by a rearrangement step at the binding interface (induced fit) [26] . This model was found to adequately describe the association kinetics of PSD-95 PDZ domain to its peptide ligands [27] . For each channel tail-PDZ pair, adequacy of the global fit was judged based on a χ 2 value smaller than 5%. In all cases, the equilibrium constant for the rearrangement step was found to be invariant of chain length as expected if such isomerization reflects a binding site rearrangement transition. The fractional co-localization of both ShA/B-C channel tail and PSD-95 proteins at the PM and in internal endosomal membrane compartments of Schneider cells ( Fig. 4 ), as well as channel clustering metrics at the whole channel level ( Fig. 5 ) were evaluated using the latest version of the Photoshop software that includes an image processing measurements module (Adobe CS6 extended version). Briefly, the co-localization yellow signal of the merged images of ~12 different cells was evaluated in both the PM and internal membrane compartments. This was achieved by sampling the yellow-marked membrane cluster signal followed by use of the ‘Grow’ and ‘Similar’ select commands until all membrane clusters were selected. Measurements of the area and perimeter of all marked clusters were then automatically recorded. For cell surface expression measurements, the overall cumulative area of all cell clusters (PM- or internal membrane-associated) was then calculated, as was the cumulative area of PM-associated clusters alone. For each cell, the fractional PSD-95-mediated Kv channel membrane surface expression was obtained by dividing the latter and former cumulative areas. The analysis above was repeated, in a blind manner, yielding similar results to those reported here. To test whether cluster area size (a dependent variable) differs between the two channel variants (an independent variable), and since the variant cluster area size distributions appear non-normal, a generalized linear model analysis was performed with Gamma distribution assumed for the cluster area size variable and log link function between the linear predictor and the mean of the distribution function. To examine whether the range and shape of the A and B cluster area size distributions differ, the respective Moses extreme reaction and Kolmogorov–Smirnov non-parametric tests were employed. How to cite this article: Zandany, N. et al . Alternative splicing modulates Kv channel clustering through a molecular ball and chain mechanism. Nat. Commun. 6:6488 doi: 10.1038/ncomms7488 (2015).